Matrix softness regulates plasticity of tumour-repopulating cells via H3K9 demethylation andSox2expression Tumour-repopulating cells (TRCs) are a self-renewing, tumorigenic subpopulation of cancer cells critical in cancer progression. However, the underlying mechanisms of how TRCs maintain their self-renewing capability remain elusive. Here we show that relatively undifferentiated melanoma TRCs exhibit plasticity in Cdc42-mediated mechanical stiffening, histone 3 lysine residue 9 (H3K9) methylation, Sox2 expression and self-renewal capability. In contrast to differentiated melanoma cells, TRCs have a low level of H3K9 methylation that is unresponsive to matrix stiffness or applied forces. Silencing H3K9 methyltransferase G9a or SUV39h1 elevates the self-renewal capability of differentiated melanoma cells in a Sox2-dependent manner. Mechanistically, H3K9 methylation at the Sox2 promoter region inhibits Sox2 expression that is essential in maintaining self-renewal and tumorigenicity of TRCs both in vitro and in vivo . Taken together, our data suggest that 3D soft-fibrin-matrix-mediated cell softening, H3K9 demethylation and Sox2 gene expression are essential in regulating TRC self-renewal. Tumour-initiating cells (TICs) are a self-renewing, highly tumorigenic subpopulation of cancer cells. They play a critical role in the initiation and progression of cancer [1] . These tumorigenic cells exhibit high chemo-resistance to conventional chemotherapeutic drug treatment and therefore are speculated to be key players in cancer relapses after chemotherapy [2] . However, the concept of TICs has been controversial. Past reports show that a high percentage (>25%) of human melanoma cells can generate a tumour in a NOD-SCID interleukin-2 receptor-γ chain null (IL2rγ −/− ) mouse [3] , [4] , suggesting that there is no hierarchy of clonal repopulation in melanoma. We recently developed a mechanical method of selecting TICs from cancer cell lines and primary cancer cells by culturing single cancer cells in soft fibrin gels [5] . Remarkably, in addition to being able to generate local primary tumours in wild-type syngeneic mice, when injected in tail veins, as few as ten of such cells can generate distant metastatic colonization and grow tumours in the lungs of wild-type non-syngeneic mice. Therefore, we functionally define these soft-fibrin-gel-selected melanoma cells as tumour-repopulating cells (TRCs) based on their high efficiency in repopulating tumours in wild-type syngeneic and non-syngeneic mice. Soon after our report, three other groups independently provide strong experimental evidence in mice that TRCs do exist in brain [6] , skin [7] and intestinal [8] tumours. In vivo imaging of unperturbed tumours further confirmed the existence of TRCs [9] , [10] . However, the underlying mechanisms of how TRCs maintain their self-renewing capability remain elusive. In the current study, we demonstrate that melanoma TRCs exhibit plasticity in mechanical stiffening, histone 3 lysine residue 9 (H3K9) methylation, Sox2 expression and self-renewal. Three-dimensional (3D) soft fibrin matrices promote H3K9 demethylation and increase Sox2 expression and self-renewal, whereas stiff ones exert opposite effects. Self-renewal plasticity of TRCs It is known that soft substrates can sustain self-renewal of mouse embryonic stem cells [11] and substrate rigidity can regulate the fate of mesenchymal stem cells [12] , indicating that rigidity of extracellular matrix plays an important role in the maintenance and regulation of stem cell properties. As TRCs are selected from a population of melanoma cells that are usually cultured on rigid plastic, we asked what would happen if we plated these TRCs back to rigid substrates. To determine the effect of substrate rigidity on the gene expression, we cultured TRCs on rigid plastic for 1, 3, 5 and 7 days, and quantified their Sox2 expression. TRCs gradually lost Sox2 expression in both mRNA and protein levels along with the culture time on plastic ( Fig. 1a,b and Supplementary Fig. 18c,d ). Sox2 expression of TRCs dramatically decreased after 1 day and was as low as that of control cells after 3 days on plastic. Other stem cell genes Bmi-1 , C-kit , Nestin and Tert , which are upregulated in TRCs [5] , were also downregulated after culture on plastic ( Supplementary Fig. 1 ). 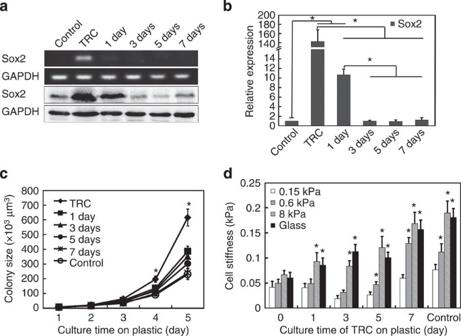Figure 1: Inhibition of Sox2 expression and self-renewal of TRCs on 2D rigid substrates. (a)Sox2expression at both mRNA level (top panel) and protein level (bottom panel). Control: B16-F1 cells cultured on plastic. TRC: Control B16-F1 cells were cultured in 90-Pa fibrin gels for 5 days. 1 day, 3 days, 5 days or 7 days: TRCs were seeded on 2D rigid dishes for 1, 3, 5 or 7 days. Images are representatives of three independent RT–PCRs and two independent western blotting experiments. (b) Quantification ofSox2expression by real time RT–PCR. Mean±s.e.m.;n=3 independent experiments. *P<0.05. (c) 2D rigid substrates inhibit TRC growth. Significant differences between Control and TRC, or 1 or 3 days from Day 1 to 5 in the 90-Pa fibrin gels (allP<0.05, except TRC at day 2, whereP=0.068, 1 day at day 2, whereP=0.52, and 3 days at Day 2 and Day 3, whereP>0.15). No differences between Control and 5 or 7 days from Day 1–5 (allP>0.06, except 5 days at Day 1 and Day 3, whereP<0.04). Each data point was averaged from at least 30 colonies. *P<0.05 between TRC and all other groups. (d) 2D rigid substrates promote stiffening of TRCs with substrate rigidity. B16-F1 cells cultured on plastic were used as a control. All were compared with ‘0.15 kPa’ in each group. Mean±s.e.m.; *P<0.01. Each data point was averaged from >150 cells from two independent experiments. All the statistics were conducted using Student’st-test throughout the manuscript unless otherwise specified. Figure 1: Inhibition of Sox2 expression and self-renewal of TRCs on 2D rigid substrates. ( a ) Sox2 expression at both mRNA level (top panel) and protein level (bottom panel). Control: B16-F1 cells cultured on plastic. TRC: Control B16-F1 cells were cultured in 90-Pa fibrin gels for 5 days. 1 day, 3 days, 5 days or 7 days: TRCs were seeded on 2D rigid dishes for 1, 3, 5 or 7 days. Images are representatives of three independent RT–PCRs and two independent western blotting experiments. ( b ) Quantification of Sox2 expression by real time RT–PCR. Mean±s.e.m. ; n =3 independent experiments. * P <0.05. ( c ) 2D rigid substrates inhibit TRC growth. Significant differences between Control and TRC, or 1 or 3 days from Day 1 to 5 in the 90-Pa fibrin gels (all P <0.05, except TRC at day 2, where P =0.068, 1 day at day 2, where P =0.52, and 3 days at Day 2 and Day 3, where P >0.15). No differences between Control and 5 or 7 days from Day 1–5 (all P >0.06, except 5 days at Day 1 and Day 3, where P <0.04). Each data point was averaged from at least 30 colonies. * P <0.05 between TRC and all other groups. ( d ) 2D rigid substrates promote stiffening of TRCs with substrate rigidity. B16-F1 cells cultured on plastic were used as a control. All were compared with ‘0.15 kPa’ in each group. Mean±s.e.m. ; * P <0.01. Each data point was averaged from >150 cells from two independent experiments. All the statistics were conducted using Student’s t -test throughout the manuscript unless otherwise specified. Full size image To examine the functional consequences of the loss of Sox2 and other stem cell genes, we re-plated those TRCs back into 90-Pa soft fibrin gels after culture on rigid substrates for 1, 3, 5 and 7 days, respectively. The growth rate of spheroids in fibrin matrices successively decreased with the culture time of TRCs on plastic ( Fig. 1c ), which is not a result of the increased apoptosis rate ( Supplementary Fig. 2 ). Moreover, colony number was also decreased ( Supplementary Fig. 3 ). After 7-day culture on plastic, TRC colonies proliferated at a similar rate as control cells (harvested from rigid dishes). The lower colony size and number suggest that rigid substrates significantly reduce the self-renewal capability of TRCs, likely due to the loss of Sox2 and other stem cell gene expressions. Besides the differences in gene expression patterns, TRCs also differ from control melanoma cells in their non-stiffening response to the increase in substrate rigidity [5] . To explore whether switching to rigid plastic may also change biophysical properties of TRCs, we first seeded them on two-dimensional (2D) rigid plastic for 1–7 days, and then quantified their stiffness on polyacrylamide (PA) gels of different rigidities. TRCs started to stiffen with substrate rigidity after 1-day culture on plastic ( Fig. 1d ). The stiffening response was more evident after 3 and 5 days. Interestingly, after 7-day culture on plastic, the stiffness and the stiffening response of TRCs were essentially the same as those of control melanoma cells ( Fig. 1d ). Regulation of H3K9 methylation by matrix and soluble factors Our data have shown major differences in self-renewal gene expression and biophysical properties between TRCs and control melanoma cells. As these two types of cells are genetically identical, we hypothesized that epigenetics may play a role in it. A large body of work has shown aberrant changes in epigenetic features during tumour initiation and progression [13] , [14] , including histone modification. Among those aberrations, H3K9 is hypermethylated in several types of tumours [15] , [16] . We asked what role H3K9 methylation plays in TRCs. To explore H3K9 methylation of TRCs, we developed a CFP-YPet H3K9 fluorescence resonance energy transfer (FRET) biosensor (fused with a nuclear localization signal (NLS)) modified from a previously reported CFP–YFP H3K9 biosensor [17] to quantify H3K9 di- and trimethylation (me2 and me3) in the nucleus of single cells ( Supplementary Fig. 4a ). This FRET probe uniquely measures the spatial distribution of H3K9 methylation level in the nucleus and revealed that H3K9 me2 and me3 mostly occurred at the nuclear periphery ( Supplementary Fig. 4b ). Culturing control cells in 90-Pa fibrin gels for merely 3 h resulted in H3K9 demethylation ( Fig. 2a ). TRCs did not elevate their H3K9 methylation (within 15 h of plating) with substrate stiffness on PA gels coated with either collagen-1 or fibrinogen ( Fig. 2b,d ); in contrast, control cells increased their H3K9 methylation with substrate stiffness on PA gels coated with collagen-1 but not with fibrinogen ( Fig. 2b,c ). Interestingly, high level of H3K9 methylation in control cells was associated with high cellular tractions on collagen-1-coated substrates and inhibition of the tractions decreased H3K9 methylation ( Supplementary Fig. 5 ), suggesting that high endogenous forces transmitted via α 1 / α 2 β 1 (collagen-1 receptor) rather than via α v β 3 (fibrinogen receptor) might be responsible for the stiff substrate-mediated H3K9 methylation, consistent with a report that activation of β 1 integrin but not β 3 integrin elevates cell traction forces [18] . 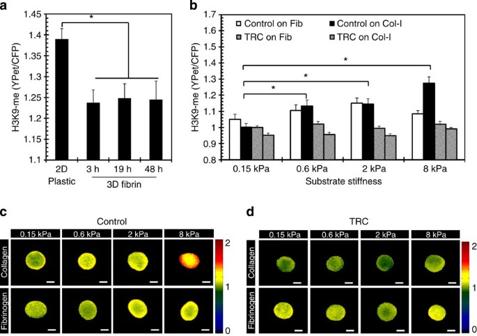Figure 2: Matrix rigidity mediated H3K9 methylation in control cells but not in TRCs. (a) H3K9 methylation is lower in 90-Pa fibrin gels than on rigid plastic. Control B16-F1 cells were transfected with the H3K9 FRET methylation biosensor and then plated either on gelatin-coated rigid plastic (2D plastic) or in the 90-Pa soft 3D fibrin gel (3D Fibrin). H3K9 methylation was measured at the indicated times after cell plating. Mean±s.e.m.;n>75 cells for each value (*P<0.001). (b) H3K9 methylation in control B16-F1 cells (Control) but not in TRCs increases on stiff PA substrates coated with collagen I (Col-1) but not fibrinogen (Fib). PA, polyacrylamide. H3K9 methylation was measured 15 h after cell plating. Mean±s.e.m.,n>40 cells for each value (*P<0.005).Representative FRET images of a cell nucleus for control cells (c) and TRCs (d) on PA gels coated with collagen I (top panel)) or fibrinogen (bottom panel). Scale bars, 5 μm. Figure 2: Matrix rigidity mediated H3K9 methylation in control cells but not in TRCs. ( a ) H3K9 methylation is lower in 90-Pa fibrin gels than on rigid plastic. Control B16-F1 cells were transfected with the H3K9 FRET methylation biosensor and then plated either on gelatin-coated rigid plastic (2D plastic) or in the 90-Pa soft 3D fibrin gel (3D Fibrin). H3K9 methylation was measured at the indicated times after cell plating. Mean±s.e.m. ; n >75 cells for each value (* P <0.001). ( b ) H3K9 methylation in control B16-F1 cells (Control) but not in TRCs increases on stiff PA substrates coated with collagen I (Col-1) but not fibrinogen (Fib). PA, polyacrylamide. H3K9 methylation was measured 15 h after cell plating. Mean±s.e.m., n >40 cells for each value (* P <0.005).Representative FRET images of a cell nucleus for control cells ( c ) and TRCs ( d ) on PA gels coated with collagen I (top panel)) or fibrinogen (bottom panel). Scale bars, 5 μm. Full size image To further explore the role of physical forces in H3K9 methylation, we applied exogenous forces via RGD (Arg-Gly-Asp)-coated magnetic beads to single cells using magnetic twisting cytometry [19] ( Fig. 3a,b ). On fibrinogen-coated stiff substrates (Glass), the applied forces induced significant increases in H3K9 methylation at the nuclear periphery within 60 min only in control cells, but not in TRCs ( Fig. 3a–c ). The force-induced H3K9 methylation was dependent on force magnitude and specifically mediated via β 1 integrin, as low forces, forces applied via beads coated with poly- L -lysine, or forces applied after blocking β 1 integrin with monoclonal antibody, was not able to induce H3K9 methylation ( Fig. 3d ). In addition, silencing H3K9 methyltransferase G9a or SUV39h1 (knockdown efficiency was ~50%; Fig. 4a ) not only reduced the baseline level of H3K9 methylation in control melanoma cells ( Fig. 4c ), but also completely blocked the force-induced H3K9 methylation ( Fig. 3d ), consistent with a report that these two enzymes are critical to H3K9 methylation [20] . In contrast, silencing or inhibiting H3K9 demethylase KDM7 with small interfering RNA (siRNA) or with Daminozide in cells in 3D soft fibrin gels increased H3K9 methylation levels ( Fig. 4b ). These data suggest that H3K9 methylation levels in these melanoma cells are controlled by both methyltransferases and demethylases. H3K9 methylation also depended on intactness of the cytoskeleton and cellular tension, as disrupting actin microfilaments with Latrunculin A or microtubules with colchicine and inhibiting myosin light chain kinase with ML7 significantly lowered H3K9 methylation levels ( Fig. 4d ). Although TRCs did not increase H3K9 methylation with substrate stiffness within 15 h ( Fig. 2b,d ), they started to increase H3K9 methylation on collagen-1-coated plastic after 48 h ( Fig. 3e ). In contrast, TRCs treated with retinoic acid (a nonspecific soluble differentiation factor) for 60 min (similar in duration for external force-induced H3K9me; see Fig. 3c ) increased H3K9 methylation levels ( Fig. 3f ), suggesting H3K9 methylation may be associated with the differentiation of TRCs. 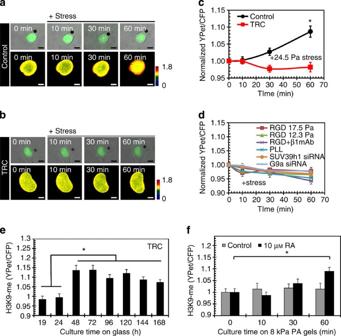Figure 3: Exogenous forces increase H3K9 methylation level via β1 integrin. Exogenous forces increase H3K9 methylation in control B16-F1 cells (a) but not in TRCs (b). Top: bright-field and fluorescence overlay image of the cells; the magnetic bead is shown as a black dot. Bottom: representative FRET images showing the spatial distribution of H3K9 methylation in the nucleus during loading. Cells were plated on 8 kPa PA gels coated with fibrinogen and loaded at 24.5 Pa, 0.3 Hz with RGD-coated ferromagnetic beads. H3K9 methylation clearly increases inaat the nuclear periphery 30–60 min after loading. Scale bars, 10 μm (top), 5 μm (bottom). (c) Quantification of H3K9 methylation inaandbduring loading. (d) No force-induced elevation of H3K9 methylation was observed when the externally applied stress magnitude was equal or <17.5 Pa, when β1integrin was blocked by a monoclonal antibody, when the force was applied via a poly-L-lysine coated bead, or when siRNA was transfected to knockdown G9a and SUV39h1, which are methyltransferases responsible for dimethylation and trimethylation of H3K9, respectively. Knockdown of G9a and SUV39h1 was confirmed by western blottings that these proteins reduced by ~50% when compared with control. (e) H3K9 methylation in TRCs increases after 2-day culture on glass dishes. TRCs were cultured on collagen I-coated glass-bottomed dishes and H3K9 methylation was measured at indicated times. Mean±s.e.m.,n>40 cells for each time point, *P<0.05. (f) Short time treatment with retinoic acid (RA) increases H3K9 methylation in TRCs. TRCs were cultured on collagen I-coated 8-kPa PA gels for 15 h. Cells were then treated with or without (Control) 10 μM RA. Note that all the values were normalized to the value at 0 min (15 h after plating). Mean±s.e.m.,n>40 cells for each value, *P<0.05. Figure 3: Exogenous forces increase H3K9 methylation level via β1 integrin. Exogenous forces increase H3K9 methylation in control B16-F1 cells ( a ) but not in TRCs ( b ). Top: bright-field and fluorescence overlay image of the cells; the magnetic bead is shown as a black dot. Bottom: representative FRET images showing the spatial distribution of H3K9 methylation in the nucleus during loading. Cells were plated on 8 kPa PA gels coated with fibrinogen and loaded at 24.5 Pa, 0.3 Hz with RGD-coated ferromagnetic beads. H3K9 methylation clearly increases in a at the nuclear periphery 30–60 min after loading. Scale bars, 10 μm (top), 5 μm (bottom). ( c ) Quantification of H3K9 methylation in a and b during loading. ( d ) No force-induced elevation of H3K9 methylation was observed when the externally applied stress magnitude was equal or <17.5 Pa, when β 1 integrin was blocked by a monoclonal antibody, when the force was applied via a poly- L -lysine coated bead, or when siRNA was transfected to knockdown G9a and SUV39h1, which are methyltransferases responsible for dimethylation and trimethylation of H3K9, respectively. Knockdown of G9a and SUV39h1 was confirmed by western blottings that these proteins reduced by ~50% when compared with control. ( e ) H3K9 methylation in TRCs increases after 2-day culture on glass dishes. TRCs were cultured on collagen I-coated glass-bottomed dishes and H3K9 methylation was measured at indicated times. Mean±s.e.m., n >40 cells for each time point, * P <0.05. ( f ) Short time treatment with retinoic acid (RA) increases H3K9 methylation in TRCs. TRCs were cultured on collagen I-coated 8-kPa PA gels for 15 h. Cells were then treated with or without (Control) 10 μM RA. Note that all the values were normalized to the value at 0 min (15 h after plating). Mean±s.e.m., n >40 cells for each value, * P <0.05. 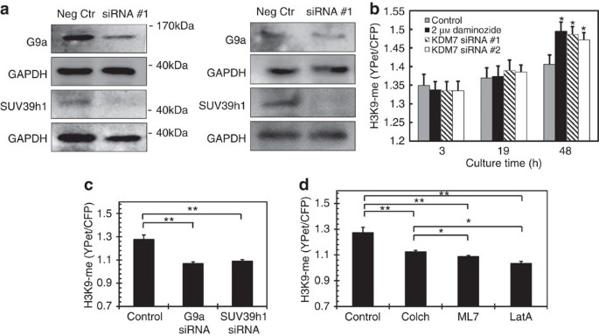Figure 4: H3K9 methylation levels depend on methyltransferases and demethylases and the tensed cytoskeleton. (a) Representative images of western blotting of G9a or SUV39h1 expression after siRNA knockdown. Control melanoma cells were transfected with two sets of G9a/SUV39h1 siRNAs (1 and 2), respectively, and western blotting assays were performed to confirm the knockdown efficiencies to be 48% (1 siRNA) and 45% (2 siRNA) for G9a, and 58% (1 siRNA) and 43% (2 siRNA), respectively. Three independent experiments showed similar results. (b) Silencing or inhibiting demethylase KDM7 increases H3K9 methylation of control melanoma cells in soft fibrin gels. Control cells were transfected with H3K9 FRET biosensors andKDM7siRNAs (1 and 2) or negative control siRNA, or treated with KDM7 inhibitor daminozide. The cells were seeded into 3D soft fibrin gels and H3K9 methylation levels were measured after 3, 19 or 48 h. Mean±s.e.m.;n>40 cells for each data point; *P<0.05. (c) Knockdown of G9a or SUV39h1 decreases the H3K9 methylation in control B16-F1 cells. (d) Inhibiting microtubule, myosin light chain kinase (MLCK) or actin polymerization decreases H3K9 methylation. Control B16-F1 cells were incubated with Colchicine (Colch, 10 μM for 30 min) to inhibit microtubule polymerization, ML7 (25 μM for 30 min) to inhibit myosin light chain kinase, or Latrunculin A (LatA, 1 μM for 30 min) to disrupt actin filaments. Mean±s.e.m;n>40 cells for each data point; *P<0.05; **P<0.001. Full size image Figure 4: H3K9 methylation levels depend on methyltransferases and demethylases and the tensed cytoskeleton. ( a ) Representative images of western blotting of G9a or SUV39h1 expression after siRNA knockdown. Control melanoma cells were transfected with two sets of G9a/SUV39h1 siRNAs (1 and 2), respectively, and western blotting assays were performed to confirm the knockdown efficiencies to be 48% (1 siRNA) and 45% (2 siRNA) for G9a, and 58% (1 siRNA) and 43% (2 siRNA), respectively. Three independent experiments showed similar results. ( b ) Silencing or inhibiting demethylase KDM7 increases H3K9 methylation of control melanoma cells in soft fibrin gels. Control cells were transfected with H3K9 FRET biosensors and KDM7 siRNAs (1 and 2) or negative control siRNA, or treated with KDM7 inhibitor daminozide. The cells were seeded into 3D soft fibrin gels and H3K9 methylation levels were measured after 3, 19 or 48 h. Mean±s.e.m. ; n >40 cells for each data point; * P <0.05. ( c ) Knockdown of G9a or SUV39h1 decreases the H3K9 methylation in control B16-F1 cells. ( d ) Inhibiting microtubule, myosin light chain kinase (MLCK) or actin polymerization decreases H3K9 methylation. Control B16-F1 cells were incubated with Colchicine (Colch, 10 μM for 30 min) to inhibit microtubule polymerization, ML7 (25 μM for 30 min) to inhibit myosin light chain kinase, or Latrunculin A (LatA, 1 μM for 30 min) to disrupt actin filaments. Mean±s.e.m; n >40 cells for each data point; * P <0.05; ** P <0.001. Full size image H3K9 demethylation-induced Sox2 expression is critical to TRC self-renewal As H3K9 methylation has been associated with inactivation of certain genes [13] , [14] , [15] , we postulated that H3K9 demethylation might be related to Sox2 expression. Our western blotting analysis showed that control cells expressed higher levels of H3K9 me2 and H3K9 me3 compared with TRCs ( Supplementary Fig. 6a ). Importantly, silencing H3K9 methyltransferase G9a or SUV39h1 in control cells significantly increased their Sox2 expression ( Fig. 5a and Supplementary Fig. 7a ), suggesting that H3K9 demethylation can increase Sox2 expression. To further investigate how H3K9 demethylation promotes Sox2 expression, we performed chromatin immunoprecipitation (ChIP) assay to quantify H3K9 me2 and me3 levels in the promoter region of Sox2 . H3K9 me2 and H3K9 me3 levels were ~50% higher in the promoter region of Sox2 in control cells than in TRCs ( Fig. 5b and Supplementary Fig. 6b ). Silencing G9a or SUV39h1 in control cells greatly decreased their H3K9-me2 or H3K9-me3 levels in the promoter region of Sox2 ( Fig. 5b ). Plating TRCs on plastic for 7 days elevated H3K9 me2 and me3 to the same levels as those in control cells ( Fig. 5b and Supplementary Fig. 6b ). These results suggest that G9a and SUV39h1 methylated H3K9 at the Sox2 promoter site blocks Sox2 expression. In contrast, TRCs did not express G9a and SUV39h1 proteins and silencing Sox2 in TRCs did not increase the expression of G9a or SUV39h1 ( Supplementary Fig. 8 ), suggesting that G9a and SUV39h1 may be independent of Sox2 expression. 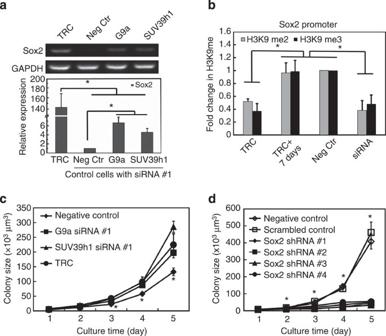Figure 5:H3K9 demethylation-mediatedSox2expression is essential forin vitrotumourgrowth. (a) Silencing G9a or SUV39h1 promotes Sox2 expression in control melanoma cells, quantified by real-time RT–PCR. Neg Ctr: negative control. *P<0.05. (b) H3K9 di- (me2) and trimethylation (me3) levels in the promoter region ofSox2quantified by the ChIP assay. TRC+7 days: TRCs were cultured on plastic for 7 days; Neg Ctr, siRNA: control melanoma cells were treated with negative control siRNA, G9a (for H3K9 me2) or SUV39h1 (for H3K9 me3) siRNA #1, respectively. *P<0.05. (c) H3K9 demethylation in control melanoma cells promotes their self-renewal capability. Control cells were transfected with G9a or SUV39h1 siRNA and then re-plated in soft fibrin gels. (d) SilencingSox2greatly inhibits growth of TRC spheroids. TRCs were transfected withSox2shRNAs or scrambled shRNA. These cells were then re-plated into 90-Pa fibrin gels. Each data point was averaged from at least 40 colonies. Inc, significant differences between Negative Control and G9a siRNA 1 or SUV39h1 siRNA 1 or TRC from day 2 to day 5 (*P<0.05, except G9a siRNA 1 at day 2, whereP=0.09). Ind, significant differences between Negative control or Scrambled control and Sox2 shRNA 1 to 4 from day 2 to day 5. (*P<0.05). Mean±s.e.m.;n=3 independent experiments for all subfigures. Figure 5: H3K9 demethylation-mediated Sox2 expression is essential for in vitro tumour growth. ( a ) Silencing G9a or SUV39h1 promotes Sox2 expression in control melanoma cells, quantified by real-time RT–PCR. Neg Ctr: negative control. * P <0.05. ( b ) H3K9 di- (me2) and trimethylation (me3) levels in the promoter region of Sox2 quantified by the ChIP assay. TRC+7 days: TRCs were cultured on plastic for 7 days; Neg Ctr, siRNA: control melanoma cells were treated with negative control siRNA, G9a (for H3K9 me2) or SUV39h1 (for H3K9 me3) siRNA #1, respectively. * P <0.05. ( c ) H3K9 demethylation in control melanoma cells promotes their self-renewal capability. Control cells were transfected with G9a or SUV39h1 siRNA and then re-plated in soft fibrin gels. ( d ) Silencing Sox2 greatly inhibits growth of TRC spheroids. TRCs were transfected with Sox2 shRNAs or scrambled shRNA. These cells were then re-plated into 90-Pa fibrin gels. Each data point was averaged from at least 40 colonies. In c , significant differences between Negative Control and G9a siRNA 1 or SUV39h1 siRNA 1 or TRC from day 2 to day 5 (* P <0.05, except G9a siRNA 1 at day 2, where P =0.09). In d , significant differences between Negative control or Scrambled control and Sox2 shRNA 1 to 4 from day 2 to day 5. (* P <0.05). Mean±s.e.m. ; n =3 independent experiments for all subfigures. Full size image As knocking down G9a or SUV39h1 can induce Sox2 expression in control cells, we further explored whether H3K9 demethylation can promote their self-renewal capability. Silencing G9a or SUV39h1 in control cells significantly increased the colony growth in soft fibrin gels to a level similar to that of TRCs ( Fig. 5c and Supplementary Fig. 7b ), but the colony number was still twofold less than that of TRCs ( Supplementary Fig. 7c,d ). However, simultaneously silencing G9a (or SUV39h1) and Sox2 completely abrogated the colony growth but not the colony number ( Supplementary Fig. 9 ), suggesting that H3K9 demethylation promotes self-renewal capability of melanoma cells in a Sox2 -dependent manner. H3K9 methylation is regulated by both methyltransferases and demethylases. Silencing KDM7, an important demethylase for H3K9 (ref. 21 ), significantly elevated H3K9 methylation ( Fig. 4b ) and suppressed colony growth and number ( Fig. 6a,b ), probably through inhibition of Sox2 expression ( Fig. 6c ). Treatment with two separate inhibitors of KDM4 (ref. 22 ) (another demethylase for H3K9) led to dose-dependent inhibition of colony size and colony number ( Supplementary Fig. 10 ). Taken together, these data suggest that H3K9 demethylation by deactivating methyltransferases or activating demethylases increases Sox2 expression and thus promotes self-renewal capability. 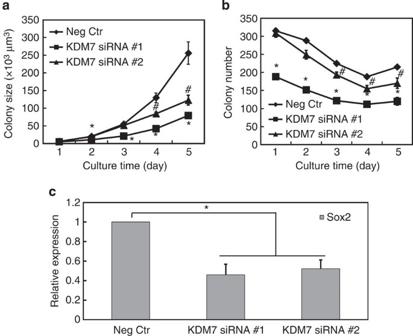Figure 6:Silencing H3K9 demethylase KDM7 greatly inhibits colony size and number through suppression ofSox2expression. Knocking down KDM7 using two different siRNAs significantly inhibits colony size (a) and number (b). Control melanoma cells were transfected with KDM7 siRNA 1 or 2, and then cultured in 90-Pa fibrin gels. Colony number was counted and colony size was monitored until day 5 (n=2). There is a significant difference between Neg Ctr and KDM7 siRNA 1 inafrom day 2 through day 5 (allP<0.00001) and inbfrom day 1 through day 5 (allP<0.01), and between Neg Ctr and KDM7 siRNA 2 in (a) at day 4 and day 5 (bothP<0.005) and inbfrom day 3 through day 5 (allP<0.05). ‘*’ and ‘#’ indicates significant differences between Neg Ctr and KDM7 siRNA 1 or 2, respectively. (c) Silencing KDM7 significantly suppressesSox2expression. Control melanoma cells were transfected with KDM7 siRNA 1 or 2, or negative control siRNA and then cultured in 90-Pa fibrin gels. After 5 days,Sox2expression was quantified by real time RT–PCR. *P<0.05;n=3 independent experiments. Figure 6: Silencing H3K9 demethylase KDM7 greatly inhibits colony size and number through suppression of Sox2 expression. Knocking down KDM7 using two different siRNAs significantly inhibits colony size ( a ) and number ( b ). Control melanoma cells were transfected with KDM7 siRNA 1 or 2, and then cultured in 90-Pa fibrin gels. Colony number was counted and colony size was monitored until day 5 ( n =2). There is a significant difference between Neg Ctr and KDM7 siRNA 1 in a from day 2 through day 5 (all P <0.00001) and in b from day 1 through day 5 (all P <0.01), and between Neg Ctr and KDM7 siRNA 2 in ( a ) at day 4 and day 5 (both P <0.005) and in b from day 3 through day 5 (all P <0.05). ‘*’ and ‘#’ indicates significant differences between Neg Ctr and KDM7 siRNA 1 or 2, respectively. ( c ) Silencing KDM7 significantly suppresses Sox2 expression. Control melanoma cells were transfected with KDM7 siRNA 1 or 2, or negative control siRNA and then cultured in 90-Pa fibrin gels. After 5 days, Sox2 expression was quantified by real time RT–PCR. * P <0.05; n =3 independent experiments. Full size image We further investigated the functional role of Sox2 in maintaining self-renewal of TRCs in vitro and in vivo . Silencing Sox2 greatly decreased the expressions of Sox2 , Bmi-1 and C-kit in TRCs ( Supplementary Fig. 11 ). Colony growth was suppressed by >90% in Sox2 -knocked down TRCs in comparison with that of control TRCs ( Fig. 5d ), suggesting that Sox2 is essential in maintaining self-renewal of TRCs in vitro . Sox2 silencing had no effects on control melanoma cells (these cells express little Sox2 ) that were grown on plastic and were then embedded in 3D stiff fibrin gels, suggesting that there were little off-target effects of Sox2 silencing ( Supplementary Fig. 12 ). Overexpressing Sox2 in control melanoma cells increased the colony number but not colony growth ( Supplementary Fig. 13 ), indicating that this intervention increases the number of self-renewing cells but does not alter cell cycle duration of a self-renewing cell. Importantly, subcutaneously injecting 100 of TRCs treated with Sox2 short hairpin RNA (shRNA) into wild-type syngeneic C57BL/6 mice did not generate any tumours by day 19. In contrast, palpable tumours were observed for untreated TRCs by day 13 and treated with scrambled control shRNA by day 15. By day 28, 2 out of 16 mice for TRCs treated with Sox2 shRNA had small tumours ( Supplementary Table 1 ), whereas for untreated TRCs 9 out of 16 mice formed large tumours; for TRCs treated with scrambled shRNA, 3 out of 8 formed tumours. The formation of tumours in TRCs treated with Sox2 shRNA appearing at late stages probably reflects the fact that the knockdown of Sox2 by shRNA was transient such that Sox2 expression came back in these cells after shRNA effect was depleted. As expected from previous findings [5] , injecting 100 of control melanoma cells (harvested from rigid plastic) did not form any tumours (0/8; Supplementary Table 1 ). These data demonstrate that Sox2 expression is necessary to sustain self-renewal capability of TRCs both in vitro and in vivo . Because of the importance of Sox2 and H3K9 demethylation in TRCs, we asked what roles Sox2 expression and H3K9 methylation might play in the selection and propagation of TRCs by soft fibrin gels. When control melanoma cells were transfected with Sox2 shRNA and cultured in 90-Pa fibrin gels, both growth and number of spheroids were inhibited ( Supplementary Fig. 14a,b ). Moreover, treatment with Daminozide, a highly selective inhibitor of KDM7, significantly inhibited TRC spheroid growth number ( Supplementary Fig. 14c,d ). Therefore, these data suggest that H3K9 demethylation-dependent regulation of Sox2 expression is important in TRC selection and propagation. Mechanism of cell stiffening with substrate stiffness To elucidate the mechanisms of the stiffening response plasticity, we examined the potential role of Cdc42 in cell stiffening because of its known role in inducing filopodia formation and cell spreading in B16-F1 melanoma cells [23] . TRCs expressed ~50% less Cdc42 than control cells; plating TRCs on plastic for 5 and 7 days increased their Cdc42 expression by ~30% and ~100%, respectively ( Fig. 7a ). Overexpression of Cdc42 in TRCs rescued the cell stiffening response with substrate rigidity ( Fig. 7b ), whereas silencing Cdc42 in control melanoma cells or in TRCs on plastic for 5 days completely abolished the stiffening response ( Fig. 7c ). Silencing Cdc42 in melanoma cells on rigid plastic downregulated H3K9 me2 but not H3K9 me3 ( Fig. 7d and Supplementary Fig. 15a,b ) and had no effects on Sox2 expression ( Supplementary Fig. 15c ), suggesting that Cdc42, cell stiffening and H3K9 methylation might be linked via tension-dependent cytoskeletal mechanotransduction, contributing to the biological plasticity of TRCs. 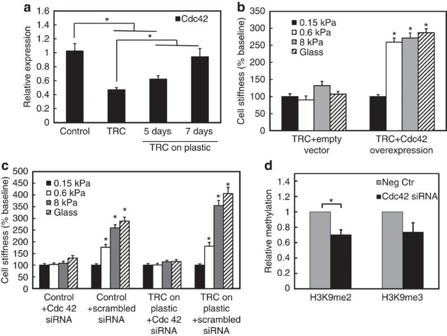Figure 7:Cdc42expression regulates stiffening response and H3K9 me2 in melanoma cells. (a) TRCs express lower level ofCdc42compared with control melanoma cells and TRCs after culture on rigid plastic for 5 or 7 days.n=6; *P<0.05; two independent experiments. (b) TRCs regain cell stiffening responses after overexpression ofCdc42. Cells were plated on Collagen-I-coated PA gels with different stiffnesses or on glass-bottomed dishes. Experiments were carried out 6 h after plating. Relative changes in cell stiffness were represented with respect to the cell stiffness on 0.15 kPa PA gel as the baseline. TRC+empty vector: TRCs were transfected with pEGFP-N1 vector; TRC+Cdc42 overexpression: TRCs were transfected withCdc42-EGFP plasmid.n>150 cells; *P<0.001. (c) Cdc42 knockdown inhibits cell stiffening in control cells and TRCs plated on plastic for 5 days. Relative changes in cell stiffness were represented with respect to the cell stiffness on 0.15 kPa PA gel as the baseline.n>100 cells; *P<0.001. Control: B16-F1 cultured on rigid plastic; TRC on plastic: TRCs were cultured on plastic for 5 days; Control+Cdc42 siRNA: control melanoma cells were transfected with Cdc42 siRNA; Control+Scrambled siRNA: control cells were transfected with scrambled siRNA; TRC on plastic+Cdc42 siRNA: TRCs were cultured on plastic for 5 days and then transfected with Cdc42 siRNA; TRC on plastic+Scrambled siRNA: TRCs were cultured on plastic for 5 days and then transfected with scrambled siRNA. Mean±s.e.m.; ‘*’ indicates significant difference compared with ‘0.15 kPa’. (d) Quantification analysis of western blotting of H3K9me2 and me3 afterCdc42knockdown in control melanoma cells. Mean±s.e.m.;n=3 independent experiments; *P<0.05. Figure 7: Cdc42 expression regulates stiffening response and H3K9 me2 in melanoma cells. ( a ) TRCs express lower level of Cdc42 compared with control melanoma cells and TRCs after culture on rigid plastic for 5 or 7 days. n =6; * P <0.05; two independent experiments. ( b ) TRCs regain cell stiffening responses after overexpression of Cdc42 . Cells were plated on Collagen-I-coated PA gels with different stiffnesses or on glass-bottomed dishes. Experiments were carried out 6 h after plating. Relative changes in cell stiffness were represented with respect to the cell stiffness on 0.15 kPa PA gel as the baseline. TRC+empty vector: TRCs were transfected with pEGFP-N1 vector; TRC+Cdc42 overexpression: TRCs were transfected with Cdc42 -EGFP plasmid. n >150 cells; * P <0.001. ( c ) Cdc42 knockdown inhibits cell stiffening in control cells and TRCs plated on plastic for 5 days. Relative changes in cell stiffness were represented with respect to the cell stiffness on 0.15 kPa PA gel as the baseline. n >100 cells; * P <0.001. Control: B16-F1 cultured on rigid plastic; TRC on plastic: TRCs were cultured on plastic for 5 days; Control+Cdc42 siRNA: control melanoma cells were transfected with Cdc42 siRNA; Control+Scrambled siRNA: control cells were transfected with scrambled siRNA; TRC on plastic+Cdc42 siRNA: TRCs were cultured on plastic for 5 days and then transfected with Cdc42 siRNA; TRC on plastic+Scrambled siRNA: TRCs were cultured on plastic for 5 days and then transfected with scrambled siRNA. Mean±s.e.m. ; ‘*’ indicates significant difference compared with ‘0.15 kPa’. ( d ) Quantification analysis of western blotting of H3K9me2 and me3 after Cdc42 knockdown in control melanoma cells. Mean±s.e.m. ; n =3 independent experiments; * P <0.05. Full size image Inhibition of TRC self-renewal by 3D stiff fibrin matrix When the cells were cultured from 2D rigid dish to 3D soft matrix, both matrix dimensionality and stiffness were altered. To further determine whether it is the 3D matrix stiffness or the effect of switching from 2D to 3D matrix that impacts on the self-renewal capability of TRCs, we cultured control B16-F1 cells in 3D soft (90-Pa) or 3D stiff (1,050-Pa) fibrin gels for 5 days. These cells were then seeded into either soft or stiff fibrin gels. After re-seeding, the cells grew better in soft fibrin gels no matter whether they were derived from soft or stiff fibrin gels; in contrast, once re-seeded in stiff fibrin gels, colony growth and number were inhibited ( Fig. 8a,b ), suggesting that switching from a 3D soft matrix to a 3D stiff matrix inhibits self-renewal and promotes quiescence of the TRCs. When culturing control melanoma cells in soft and stiff fibrin gels, a 10-fold increase in substrate stiffness leads to a ~1.25-fold increase in H3K9 me2 and a 50% increase in H3K9 me3 on the protein level, and a ~90% decrease in Sox2 expression ( Fig. 9 ). Importantly, switching from a stiff matrix (1,050-Pa) to a soft matrix (90-Pa) significantly decreased H3K9 methylation and elevated Sox2 expression by ~5-fold ( Fig. 8c,d ). Taken together, these data suggest that 3D stiff fibrin matrix can inhibit TRC self-renewal via H3K9 methylation-mediated Sox2 suppression. 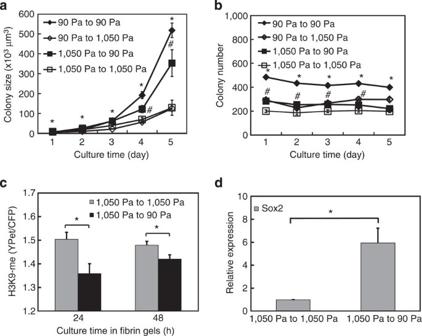Figure 8: Stiff matrix inhibits self-renewal of TRCs. Stiff fibrin gels inhibit colony growth (a) and number (b). ‘90-Pa to 90-Pa’ and ‘90-Pa to 1,050-Pa’: control B16-F1 cells were cultured in 90-Pa fibrin gels for 5 days and these cells were then re-plated into 90-Pa and 1,050-Pa fibrin gels, respectively. ‘1,050-Pa to 90-Pa’ and ‘1,050-Pa to 1050-Pa’: control B16-F1 cells were cultured in 1050-Pa fibrin gels for 5 days and these cells were then re-plated into 90-Pa or 1,050-Pa fibrin gels. Spheroid size and number were measured from Day 1 through Day 5. Inaandb, significant differences between ‘90-Pa to 90-Pa’ and ‘90-Pa to 1,050-Pa’ from Day 1 through Day 5 (allP<0.01); significant differences between ‘1,050-to 90-Pa’ and ‘1,050-Pa to 1050-Pa’ at day 4 and day 5 ina(bothP<0.02) and from day 1 to day 4 inb(allP<0.05). Mean±s.e.m.;n=2 independent experiments. Each data point was averaged from >30 colonies. ‘*’ and ‘#’ indicates significant differences between ‘90-Pa to 90-Pa’ and ‘90-Pa to 1,050-Pa’ and between ‘1,050-to 90-Pa’ and ‘1,050-Pa to 1050-Pa’, respectively. (c) Switching to 3D soft matrix decreases H3K9 methylation. Mean±s.e.m.;n>50 cells from two independent experiments; *P<0.05. (d) Switching to 3D soft matrix increasesSox2expression. Mean±s.e.m.;n=3 independent experiments; *P<0.05. Incandd, control cells were cultured in 1,050-Pa fibrin gels for 5 days and then re-plated into 90-Pa or 1,050-Pa gels. After 24 or 48 h incand 5 days ind, their H3K9 methylation was measured by FRET andSox2 expression was quantified by real time RT–PCR. Figure 8: Stiff matrix inhibits self-renewal of TRCs. Stiff fibrin gels inhibit colony growth ( a ) and number ( b ). ‘90-Pa to 90-Pa’ and ‘90-Pa to 1,050-Pa’: control B16-F1 cells were cultured in 90-Pa fibrin gels for 5 days and these cells were then re-plated into 90-Pa and 1,050-Pa fibrin gels, respectively. ‘1,050-Pa to 90-Pa’ and ‘1,050-Pa to 1050-Pa’: control B16-F1 cells were cultured in 1050-Pa fibrin gels for 5 days and these cells were then re-plated into 90-Pa or 1,050-Pa fibrin gels. Spheroid size and number were measured from Day 1 through Day 5. In a and b , significant differences between ‘90-Pa to 90-Pa’ and ‘90-Pa to 1,050-Pa’ from Day 1 through Day 5 (all P <0.01); significant differences between ‘1,050-to 90-Pa’ and ‘1,050-Pa to 1050-Pa’ at day 4 and day 5 in a (both P <0.02) and from day 1 to day 4 in b (all P <0.05). Mean±s.e.m. ; n =2 independent experiments. Each data point was averaged from >30 colonies. ‘*’ and ‘#’ indicates significant differences between ‘90-Pa to 90-Pa’ and ‘90-Pa to 1,050-Pa’ and between ‘1,050-to 90-Pa’ and ‘1,050-Pa to 1050-Pa’, respectively. ( c ) Switching to 3D soft matrix decreases H3K9 methylation. Mean±s.e.m. ; n >50 cells from two independent experiments; * P <0.05. ( d ) Switching to 3D soft matrix increases Sox2 expression. Mean±s.e.m. ; n =3 independent experiments; * P <0.05. In c and d , control cells were cultured in 1,050-Pa fibrin gels for 5 days and then re-plated into 90-Pa or 1,050-Pa gels. After 24 or 48 h in c and 5 days in d , their H3K9 methylation was measured by FRET and Sox 2 expression was quantified by real time RT–PCR. 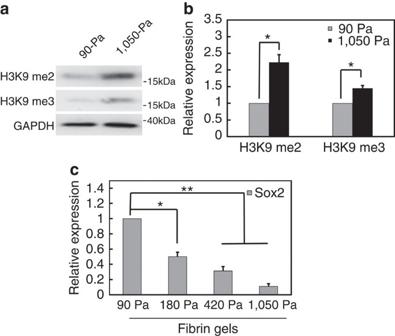Figure 9: Stiff fibrin matrix elevates H3K9 methylation levels and suppressesSox2expression. (a,b) Stiff fibrin matrix increases H3K9 methylation. Control cells were cultured in 90-Pa or 1,050-Pa fibrin gels for 5 days. Their H3K9 methylation level was analysed by western blotting assay (a) and quantified inb. (c) Stiff fibrin matrix suppressesSox2expression. Control B16-F1 cells were cultured in fibrin gels with the indicated stiffness for 5 days and then analysed forSox2expression by real-time RT-PCR. Mean±s.e.m.;n=3 independent experiments. *P<0.05; **P<0.01. Full size image Figure 9: Stiff fibrin matrix elevates H3K9 methylation levels and suppresses Sox2 expression. ( a , b ) Stiff fibrin matrix increases H3K9 methylation. Control cells were cultured in 90-Pa or 1,050-Pa fibrin gels for 5 days. Their H3K9 methylation level was analysed by western blotting assay ( a ) and quantified in b . ( c ) Stiff fibrin matrix suppresses Sox2 expression. Control B16-F1 cells were cultured in fibrin gels with the indicated stiffness for 5 days and then analysed for Sox2 expression by real-time RT-PCR. Mean±s.e.m. ; n =3 independent experiments. * P <0.05; ** P <0.01. Full size image Increasing evidence has demonstrated that TRCs truly exist as a highly tumorigenic subpopulation that is critical to tumour initiation and progression. TRCs also exhibit high resistance to conventional chemotherapeutic drug treatment, which has been speculated to drive cancer relapse after chemotherapy. Therefore, TRCs may be one of the pivotal targets to achieve complete tumour eradication [24] . In the present study, we investigated how TRCs maintain their self-renewal capability. As TRCs appear to be less differentiated, we set out to determine their specific lineage. Our data show that TRCs exhibited Sox2 high Mitf low phenotype and control melanoma cells exhibited Sox2 − Mitf + phenotype ( Supplementary Fig. 16a,b ), consistent with published results [25] , [26] , [27] and suggesting that TRCs resemble melanoblasts that are Sox2 low Mitf low and control melanoma cells resemble melanocytes that are Sox2 − Mitf + in these two gene expression patterns [27] . However, expression of Mitf upstream regulators, Pax3 (ref. 28 ) and Sox10 (ref. 27 ), and melanocyte-specific genes, tyrosinase-related protein 1 ( Tyrp1 ) [28] , dopachrome tautomerase ( DCT ) [28] and glycoprotein non-metastatic melanoma protein B ( Gpnmb ) [29] , was similar in TRCs as in control cells ( Supplementary Fig. 16c,d ). These findings suggest that melanoma TRCs may be progenitor cells of control B16-F1 cells but more differentiated than melanoblasts. Moreover, knocking down Sox2 in TRCs increased Mitf expression ( Supplementary Fig. 17a ), while silencing Mitf (knockdown efficiency ~80%; Supplementary Fig. 17b ) in control melanoma cells did not affect Sox2 expression ( Supplementary Fig. 17c ), suggesting that self-renewal gene Sox2 is independent of Mitf . Importantly, when TRCs are plated on the rigid dish, expression of melanocyte-related gene Mitf gradually increased ( Supplementary Fig. 18 ), demonstrating Mitf plasticity of TRCs when substrate rigidity was elevated, opposite in direction as the plasticity of Sox2 expression (see Fig. 1a,b ). Sox2 is known for its critical role in the maintenance of pluripotency [25] and fate determination [30] of stem cells. Sox2 also sustains self-renewal capability of TICs [26] . Inhibition or silencing of Sox2 leads to loss of tumorigenicity [26] , [31] . Sox2 dysfunction in cancer [32] , [33] is known, but it is not clear what triggers Sox2 expression in cancer. Our current study reveals a critical role of the mechanics of 3D matrix in Sox2 expression in a subpopulation of tumour cells. Importantly, silencing Sox2 greatly inhibits spheroid growth in vitro and tumour generation in vivo . TICs are heterogeneous in terms of their transient, long-term, or delayed-contributing effects on tumour growth [34] . Although we cannot exclude the possibility that TRCs isolated from soft fibrin matrices are also heterogeneous, our previous finding that as few as ten of these TRCs are sufficient to generate local and distant tumours [5] suggests that these TRCs are distinct from those TICs. Cancer cells exhibit aberrant epigenetic features, including global changes in DNA methylation and altered histone modification [35] . On the other hand, stem cells have an open chromatin structure and abnormal epigenetic regulation may be prone to malignant transformation [36] . Here we show that H3K9 demethylation by silencing G9a or SUV39h1 can greatly promote the self-renewal capability of control melanoma cells in a Sox2 -dependent manner, whereas silencing H3K9 demethylases inhibits self-renewal. It should be noted that in contrast to the increase in TRC colony number and growth observed following culture in soft substrates, silencing H3K9 methyltransferases has significant functional effects on colony growth but not colony number and the levels of Sox2 remain 30- to 40-fold lower than those found in TRCs. The exact mechanism is not clear at this time, but it may be partly due to the fact that only 50% of G9a/SUV39h1 is knocked down, whereas there are no detectable levels of G9a/SUV39h1 in TRCs ( Supplementary Fig. 8 ) and/or other self-renewal promoting effects of silencing G9a/SUV39h1 are at work. In addition, it is not clear why silencing Sox2 , overexpressing Sox2 , or inhibiting KDM4, has different effects from silencing methyltransferases on colony number and size. These issues need to be investigated in the future by dissecting out specific signalling pathways. Nevertheless, our data suggest that H3K9 demethylation and methylation, modulated by force-induced chromatin remodelling mediated by the cytoskeleton, can regulate Sox2 expression and play important roles in self-renewal and differentiation of TRCs. Our results show that stiff matrix induced H3K9 methylation occurs at the nuclear periphery just under the nuclear envelope. The applied stress (via the magnetic bead) on the cell surface via integrins also induces H3K9 methylation at the periphery of the nucleus, suggesting that stiff matrix-induced H3K9 methylation may be (at least) in part due to the elevation of endogenous stresses in the cell. These findings are in line with a recent report that force-induced stiffening of isolated nuclei depends on an intact LINC (linker of nucleoskeleton and cytoskeleton) pathway [37] . Cdc42 silencing decreases H3K9me2 by ~20%, similar to that after disruption of cytoskeletal filaments with drugs ( Fig. 4d ), suggesting that the effect of silencing Cdc42 might be important in altering cell functions. However, silencing Cdc42 has no effect on H3K9me3 or Sox2 , suggesting that some molecule(s) upstream of Cdc42 may be important in controlling H3K9me3 and Sox2 . Furthermore, our current findings suggest that increasing matrix rigidity affect Cdc42-mediated cell stiffening, H3K9 methylation and Sox2 suppression, but whether these are independent or linked pathways in controlling TRC function remains unclear and requires additional experiments in the future. Published reports suggest that G9a/SUV39h1-mediated H3K9 methylation contributes to cancer initiation and/or progression [13] , [14] , [16] , [38] , [39] , different from our findings that G9a or SUV39h1 knockdown leads to Sox2 expression. This discrepancy may lie in the fact that in those previous studies differentiated cancer cells are assayed, whereas in our present study TRCs are analysed. Although there are reports on Sox2 expression in several types of undifferentiated tumour cells [26] , [31] , there is, to the best of our knowledge, no report of H3K9 methylation or Sox2 expression in TRCs when mechanical microenvironment is perturbed. Therefore, our findings on low force-mediated H3K9 demethylation and thus Sox2 gene expression are novel. Furthermore, we find that H3K9 methylation can directly inhibit Sox2 expression. Nevertheless, the potential roles of other histone modifications, such as H3K4 and/or H3K27 methylation, acetylation and phosphorylation, and DNA methylation, remain to be elucidated. In addition, the mechanisms of in vivo Sox2 expression/suppression with the link to H3K9 demethylation/methylation and matrix compliance/cell stiffening need to be investigated in the future. We show that a uniform stiff fibrin gel functions as a physical barrier to prevent the formation and growth of TRC spheroids through elevated H3K9 methylation-induced Sox2 suppression, supporting a recent postulate on breast cancer progression [40] . Melanoma cells in the same soft fibrin gels can form round colonies only at z -heights far away from the rigid plastic bottom ( Supplementary Fig. 19 ); as these cells experience the same porosity but different elasticity, these data demonstrate that it is matrix stiffness but not porosity that dictates round colony generation and self-renewal. Furthermore, addition of soluble fibrinogen ligands to the 90-Pa fibrin matrix (total ligand amount is equivalent to that of 1,050-Pa fibrin gels) did not alter colony growth ( Supplementary Fig. 20 ), suggesting that the difference in colony growth between 90-Pa and 1,050-Pa fibrin gels may not be due to ligand density availability. It is noteworthy that the H3K9 methylation results and the corresponding traction data (and their inhibition by myosin light chain kinase inhibitor ML7) suggest that different integrin subsets (that is, collagen-1-mediated β1 integrin binding versus fibrinogen-mediated β3 integrin binding) can trigger different responses in H3K9 methylation even for the same substrate stiffness. Our data suggest that TRCs may have different cell fates in matrices of various mechanical and biochemical microenvironments ( Fig. 10 ). In a soft matrix, TRCs can proliferate well and grow into a local tumour. In the presence of soluble differentiation factors, TRCs cannot proliferate even in soft matrix. In contrast, a stiff matrix restricts TRC growth and makes them quiescent. However, on matrix degradation and remodelling, the stiff matrix may become locally softened, reactivating TRCs to proliferate, while some areas of local stiffening may promote TRCs to differentiate. Locally switching from 3D stiff matrices to 3D soft matrices and vice versa may be able to regulate TRC self-renewal, as suggested by our current results from in vitro culture. This scenario may partially explain why tumour relapses several years after surgery and therapies. These data indicate that stiff matrix may be used as an effective strategy to suppress self-renewal of TRCs. 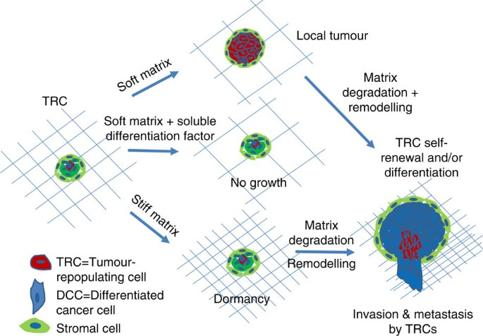Figure 10:A working model of melanomatumourgrowth and metastasis. TRCs proliferate in a soft matrix and eventually grow into a local tumour, while a stiff matrix restricts their proliferation and makes TRCs dormant. TRCs in the soft matrix can invade and self-renew and/or differentiate when the matrix is degraded and remodeled. When a soluble differentiation factor like retinoic acid is present, TRCs lose their proliferative property and stay quiescent even in soft matrix. However, on matrix degradation, the dormant TRCs in the original stiff matrix start to self-renew in weakened and soft sites and to differentiate in remodelled and stiffened sites, leading to invasion and eventual metastatic colonization by TRCs in very soft tissues/organs with rigidity of ~100 Pa, similar to those undifferentiated TRCs. It is known that majority of metastases from many types of solid tumours is found in very soft organs/tissues such as the lung, brain, liver and bone marrow45, but the underlying mechanism of this metastatic tropism is not understood. As the bone marrow stiffness is ~100 Pa (ref.54), brain stiffness is ~200–1,000 Pa (ref.54), liver stiffness is ~400 Pa (ref.55) and lung stiffness is 100–1,000 Pa (ref.56), all being very soft tissues, it is tempting to speculate that our model could be extended to metastases by other types of solid tumours, with implications in providing possible partial explanation to the conundrum of metastatic tropism. Clearly, this working model needs to be tested rigorously in the future. Figure 10: A working model of melanoma tumour growth and metastasis. TRCs proliferate in a soft matrix and eventually grow into a local tumour, while a stiff matrix restricts their proliferation and makes TRCs dormant. TRCs in the soft matrix can invade and self-renew and/or differentiate when the matrix is degraded and remodeled. When a soluble differentiation factor like retinoic acid is present, TRCs lose their proliferative property and stay quiescent even in soft matrix. However, on matrix degradation, the dormant TRCs in the original stiff matrix start to self-renew in weakened and soft sites and to differentiate in remodelled and stiffened sites, leading to invasion and eventual metastatic colonization by TRCs in very soft tissues/organs with rigidity of ~100 Pa, similar to those undifferentiated TRCs. It is known that majority of metastases from many types of solid tumours is found in very soft organs/tissues such as the lung, brain, liver and bone marrow [45] , but the underlying mechanism of this metastatic tropism is not understood. As the bone marrow stiffness is ~100 Pa (ref. 54 ), brain stiffness is ~200–1,000 Pa (ref. 54 ), liver stiffness is ~400 Pa (ref. 55 ) and lung stiffness is 100–1,000 Pa (ref. 56 ), all being very soft tissues, it is tempting to speculate that our model could be extended to metastases by other types of solid tumours, with implications in providing possible partial explanation to the conundrum of metastatic tropism. Clearly, this working model needs to be tested rigorously in the future. Full size image Published reports have shown that tension-dependent matrix stiffening is critical in breast cancer progression [41] , [42] , [43] . At a first look, it appears that there is a discrepancy in our findings and the results of these reports. A close examination reveals that our findings and theirs may be referring to different cancer cells at different stages during cancer progression. It is known that tissue stiffening alone cannot drive mammary epithelial transformation without ErbB2 activation [43] . It is possible that integrin-mediated, tension-dependent matrix stiffening facilitates differentiation and invasion of those TRCs only in the presence of matrix degradation by various proteases [42] that generate more porous matrices of heterogeneous rigidity. This explanation is supported by the experimental finding that matrix metalloproteinease 14-mediated local softening of the invasive front of mammary epithelial cells is necessary to overcome the stiff elastic resistance of the collagen matrix [44] . As tens of thousands of cancer cells differentiate on the stiff matrix, invade and then intravasate, few undifferentiated or partially differentiated cancer cells such as TRCs may follow these differentiated cancer cells and disseminate into the blood vessel. It is possible that only these soft TRCs can survive the distant organs to form metastatic colonization, the major rate-limiting step in clinically detectable macroscopic metastasis [45] . This interpretation may explain why metastatic colonization is such a highly inefficient process, with only ~0.01% intravasated cancer cells being able to form metastatic colonization [45] . The model that soft TRCs that are much softer than differentiated cancer cells and that are the key players in metastatic colonization is supported by a recent report that the core of human breast tumour tissues is much softer than peripheral tumour tissues and that metastatic tumour tissues in mouse lungs are much softer than surrounding normal lung tissues [46] . This soft cancer cell model is also supported by numerous reports over the last two decades from several labs that cancer cells, especially those metastatic cancer cells, are much softer than normal cells or non-metastatic cancer cells [47] , [48] , [49] , [50] , [51] , [52] . The long period of latency of disseminated carcinoma cells observed clinically [45] might be partially explained by the dormancy of the TRCs inside the uniformly stiff matrix, which restrains them from proliferating. This postulate needs to be tested in the future in animal models. Cell culture Murine melanoma cell line B16-F1 was purchased from American Type Culture Collection. Briefly, cells were cultured on rigid dishes with DMEM cell culture medium supplemented with 10% fetal bovine serum (Invitrogen), 2 mM L -glutamine (Invitrogen), 1 mM sodium pyruvate and 0.1 mM penicillin/streptomycin at 37 °C with 5% CO 2 . Cells were passaged every 3–4 days using TrypLE (Invitrogen). Glass or plastic culture dishes were coated with collagen-1 (0.2 mg ml −1 ) or sometimes with gelatin (0.1%) (denatured collagen) unless otherwise specified. 3D fibrin gel preparation Salmon fibrinogen and thrombin were purchased from Reagent Proteins (CA, USA). Three-dimensional fibrin gels were prepared as described previously [5] . In brief, fibrinogen was diluted into 2 mg ml −1 with T7 buffer (pH 7.4, 50 mM Tris, 150 mM NaCl). Cells were detached from 2D rigid dishes and cell density was adjusted to 10 4 cells per ml. Fibrinogen and cell solution mixture was made by mixing the same volume of fibrinogen solution and cell solution, resulting in 1 mg ml −1 fibrinogen and 5,000 cells per ml in the mixture (for 2, 4, 8 mg ml −1 (180, 420 or 1,050 Pa, respectively) fibrin gels, the initial concentration was increased to 4, 8 or 16 mg ml −1 ). Two hundred and fifty microlitres of cell/fibrinogen mixture was seeded into each well of 24-well plate and mixed well with pre-added 5 μl thrombin (100 U ml −1 ). The cell culture plate was then incubated in 37 °C cell culture incubator for 10 min. Finally, 1 ml of DMEM medium containing 10% fetal bovine serum and antibiotics was added. Reverse transcription-PCR and real-time RT–PCR analysis Total mRNA was isolated from the cells using the Trizol reagent according to the supplier’s instruction (Invitrogen). Reverse transcription (RT) was performed using the TransScript First-strand cDNA Synthesis SuperMix (TransGen), according to the manufacturer’s protocol. RT–PCR was performed using a PCR kit (QIAGEN), and real-time RT–PCR was performed using GoTaq qPCR Master Mix (Promega). The data were normalized against mouse glyceraldehyde 3-phosphate dehydrogenase. The sequences of all the primers for RT–PCR and real time RT–PCR were listed in Supplementary Tables 2 and 3 . Chromatin immunoprecipitation assay We performed ChIP assay following the manufacturer’s instructions (ChIP Assay Kit, Millipore). Briefly, cells were subjected to cross-linking with 1% formaldehyde in medium for 10 min at 37 °C and then lysed in SDS buffer for 10 min on ice. Chromatin was sonicated to shear DNA to an average length of 0.2–1.0 kb. Antibodies to di- and trimethyl histone H3 (Lys9) (Abcam) were used for immunoprecipitation. Normal mouse IgG (Santa Cruz) was used as negative control. The immunoprecipitation was heated to reverse the formaldehyde cross-linking and the DNA fragments in the precipitates were purified by phenol/chloroform extraction and ethanol precipitation. The immunoprecipitated DNA was quantified by real-time RT-PCR. Primers were sets corresponding to Sox2 and glyceraldehyde 3-phosphate dehydrogenase (negative control) promoter regions. The sequences of these promoter regions were listed in Supplementary Table 4 and can be found in Transcriptional Regulatory Element Database (Cold Spring Harbor Laboratory). Western blotting assay To quantify the expression levels of G9a, SUV39h1, H3K9 di- and trimethylation, cells were lysed with 200 μl Laemmli sample buffer (Beyotime). Twenty microlitres of each sample were separated by 8–15% SDS–PAGE, blocked with 5% BSA overnight at 4 °C and incubated with primary antibodies to G9a (Rabbit, 1:1,000, Cell Signalling, 3306), SUV39h1 (Rabbit, 1:1,000, Cell Signalling, 8729), H3K9 di-methylation (Rabbit, 1:300, Millipore, 17–648) and trimethylation (Rabbit, 1:300, Millipore, 17–625) and GAPDH (Mouse, 1:1,000, Abcam, ab8245) for 2 h at room temperature. Primary antibodies were detected with goat anti-Rabbit IgG-HRP (1:2,000, Santa Cruz, sc-2004) or anti-Mouse IgG-HRP(, 1:2,000, Santa Cruz, sc-2005). The blots were developed using SuperSignal West Pico chemiluminescent substrate (Millipore). FRET probe gene construction and plasmids The plasmid of histone H3K9 methylation reporter (ID 22866) is purchased from Addgene (Cambridge, MA). In brief, it includes a central fragment consisting of the methyl-lysine binding domain of HP1 protein and a histone peptide, which was further fused in between an amino-terminal CFP and a carboxy-terminal YFP [17] . This plasmid was digested with Bam HI and Sac I, and fused to predigested pRsetB (Invitrogen) containing C-terminal YPet and NLS. The reporter containing NLS was further digested and inserted into pcDNA3 (Invitrogen) to create modified histone methylation reporter for mammalian cell expression. The insert was sequenced (W. M. Keck Center for Functional and Comparative Genomics, University of Illinois at Urbana–Champaign) to verify the integrity of the coding sequence. FRET reporter was transfected into the cells using Lipofectamine 2000 (Invitrogen) according to manufacturer’s protocols. Magnetic twisting cytometry Magnetic twisting cytometry has been described elsewhere [19] , [53] . RGD-coated or poly- L -lysin-coated ferromagnetic beads (Fe 3 O 4 , 4 μm in diameter) were added to cells and then incubated for 30 min to allow for integrin binding and clustering. Beads were then magnetized in horizontal direction by applying a strong magnetic pulse (1,000 Gauss for 100 μs). A sinusoidal oscillatory waveform was applied at 0.3 Hz for 1 h to the apical surface of the cell. The amplitude of the magnetic field was varied at 35, 50 and 70 Gauss corresponding to 11, 15.9 and 22.2 Pa applied stress. The apparent applied stress is defined as the ratio of the applied torque to six times the bead volume and equals the bead constant times the applied twisting field. Cells were plated on collagen-coated (0.2 mg ml −1 ) or fibrinogen-coated (0.2 mg ml −1 ) PA gels with different rigidities or glass/plastic. Stiffness was quantified 6 h later. Cells were maintained in CO 2 -independent medium supplemented with 10% serum (Invitrogen) at 37 °C during experiments. A Leica inverted microscope integrated with the magnetic twisting cytometry device and Dual-View system (Optical Insight) was used to simultaneously apply stress and capture CFP and YFP (YPet) emission images. For emission ratio imaging, the Dual-View MicroImager (Optical Insights) was used. CFP/YFP Dual EX/EM (FRET) (OI-04-SEX2) has the following filter sets: CFP: excitation, S430/25, emission S470/30; YFP: excitation, S500/20, emission S535/30. The emission filter set uses a 515-nm dichroic mirror to split the two emission images. Cells were illuminated with a 100-W Hg lamp. For FRET imaging, each CFP (1,344 pixels × 512 pixels) and each YFP image (1,344 pixels × 512 pixels) were simultaneously captured on the same screen by using a charge-coupled device camera (C4742–95-12ERG; Hamamatsu) and a × 40, 0.55 numerical aperture air-immersion objective. A customized Matlab (Mathworks) programme was used to analyse CFP and YFP images and to obtain YFP/CFP emission ratio. RNA interference Cells were transfected with siRNA or shRNA, or complementary DNA using Lipofectamine 2000 (Invitrogen) following the manufacturer’s protocol. Silencer Negative Control No. 1 siRNA (Invitrogen, AM4611) was used a control in RNAi experiment. The construct sequence is 5′-GGUGAUCCUUAUGCUGUU-3′ Att for G9a siRNA 1 (Invitrogen, 90322), 5′-GGUGACUUCAGAUGUGGCCtt-3′ for G9a siRNA 2 (Invitrogen, 90133), 5′-GGUCCUUUGUCUAUAUCAAtt-3′ for SUV39h1 1 (Invitrogen, 69566), 5′-GGUGUACAACGUAUUCAUAtt-3′ for SUV39h1 2 (Invitrogen, 151927) and 5′-AGUACUGCUUACGAUACGGtt-3′ for negative control siRNA. KDM7 siRNA 1 (Santa Cruz, sc-146320) is a pool of three different siRNA duplexes, sc-146320A, sc-146320B and sc-146320C, the sequence of which is 5′-GUAGUAUACCGCAGCUUAAtt-3′, 5′-GUGAAUGGUUAGCAAUACAtt-3′ and 5′-GAGAAUGUCUCGCCUUUCAtt-3′, respectively. The sequence of KDM7 siRNA 2 is 5′-GAAAUAACAUCACACUUUAtt-3′ (Invitrogen, 503916). Mitf siRNA was purchased from Invitrogen (155366) and the construct sequence is 5′-GGUAUGAACACGCACUCUCtt-3′. Cdc42 siRNA was acquired from Invitrogen (catalogue number 66023) and the construct sequence is 5′-GGGCAAGAGGAUUAUGACAtt-3′. Sox2 shRNAs were obtained from Origene (TG515613). The construct sequence is 5′-GCACTACCAGAGCTAACTCAGATAGTACT-3′ for scrambled shRNA, 5′-GTATAACATGATGGAGACGGAGCTGAAGC-3′ for shRNA 1, 5′-AGACGCTCATGAAGAAGGATAAGTACACG-3′ for shRNA 2, 5′-AGCTACGCGCACATGAACGGCTGGAGCAA-3′ for shRNA 3, and 5′-AACATGATGGAGACGGAGCTGAAGCCGCC-3′ for shRNA 4. The Sox2 cDNA was obtained from Origene (MG204615). The Cdc42 -EGFP plasmid (ID 12975) was purchased from Addgene. pEGFP-N1 vector (Clotech) was used as control. Traction measurement. We followed the protocols of cell-traction quantification published previously [11] . In brief, cells were plated on PA gels with red fluorescent beads (0.2 μm in diameter; Molecular Probes, Invitrogen) embedded on the top surface. Before and after cell trypsinization, fluorescent images were taken to compute the displacement field of the beads using digital image correlation (DIC)in a homebuilt MATLAB program. Cell tractions were then calculated from the displacement field using inverse Boussinesq mathematical model. Mice experiments Four-week-old female C57BL/6 mice were purchased from Wuhan University Center for Animal Experiment. All animals had received humane care in compliance with the Principles of Laboratory Animal Care Formulated by the National Society of Medical Research and the guide for the National Institutes of Health of USA. The protocol was approved by the Animal Care and Use Committee of Wuhan University. B16-F1 cell spheroids were selected from 3D 90-Pa fibrin gels and pipetted to single cells. These TRCs were then transfected with Sox2 shRNA or scrambled control via Lipofectamine 2000 (Invitrogen) following the manufacturer’s protocol. These cells were harvested and the cell number was counted under microscopy. The cells were then suspended in a 0.9% NaCl solution with appropriate cell density. One hundred of TRCs transfected with Sox2 shRNA or scrambled control were subcutaneously inoculated or intravenously injected into the tail vein of wild-type C57BL/6 mice. The tumour growth of injected mice was carefully monitored every day. Colony number assay By changing the focal planes along the z axis (the direction of gel depth), the colony number was counted view by view. At least three wells of colonies were counted per condition per day. Statistical analysis All statistics (except the Fisher’s exact test for analyses of mice experiments) were performed using a two-tailed Student’s t -test. How to cite this article: Tan, Y. et al . Matrix softness regulates plasticity of tumour-repopulating cells via H3K9 demethylation and Sox2 expression. Nat. Commun. 5:4619 doi: 10.1038/ncomms5619 (2014).